Triple-helical nanowires by tomographic rotatory growth for chiral photonics Three dimensional helical chiral metamaterials resulted in effective manipulation of circularly polarized light in the visible infrared for advanced nanophotonics. Their potentialities are severely limited by the lack of full rotational symmetry preventing broadband operation, high signal-to-noise ratio and inducing high optical activity sensitivity to structure orientation. Complex intertwined three dimensional structures such as multiple-helical nanowires could overcome these limitations, allowing the achievement of several chiro-optical effects combining chirality and isotropy. Here we report three dimensional triple-helical nanowires, engineered by the innovative tomographic rotatory growth, on the basis of focused ion beam-induced deposition. These three dimensional nanostructures show up to 37% of circular dichroism in a broad range (500–1,000 nm), with a high signal-to-noise ratio (up to 24 dB). Optical activity of up to 8° only due to the circular birefringence is also shown, tracing the way towards chiral photonic devices that can be integrated in optical nanocircuits to modulate the visible light polarization. Advanced chiral photonic components that are able to manipulate the polarization state of light are widely required in several application fields [1] , [2] , [3] , [4] , [5] . Recently, chiral metamaterials have attracted great interest because of the possibility to achieve negative refraction by means of chirality [6] or to artificially reproduce and enhance the weak chiro-optical effects present in natural chiral molecules (enantiomers). Indeed, quasi-free electrons in collective plasmon oscillations have been shown to overcome some natural limitations in two-dimensional chiral metamaterial structures [7] , [8] , [9] . However, these structures need oblique incidence of light to discriminate polarizations with opposite handedness and also exhibit weak dichroic selection. To maximize the interaction with light, chiral metamaterials should extrude along the third dimension, that is, by a stacked arrangement of a unit cell (quasi-three-dimensional (3D) objects) [10] , [11] , [12] , [13] , [14] , [15] . In particular, fully 3D helix-based metamaterials can be considered as the best candidates for pronounced chiral response integrated in compact devices, as demonstrated by the fully 3D helical metamaterials acting as circular polarizers in the infrared range [2] , and realized by direct laser writing. Most recently, the development of bottom-up technologies, based on block copolymer self-assembly followed by electrodeposition, has allowed the realization of nanoplasmonic gyroid metamaterial [16] . In this particular structure, the presence of a network of multiple interconnected helical wires with opposite handedness provides 3D chirality in the visible range [17] , which has been explained by a simplified 3D-oriented helical metamaterial model [18] , [19] . These results suggest further exploitation of this chiral geometry towards the achievement of additional, integrated, chiro-optical properties such as broadband circular dichroism (CD) in the visible range, high signal-to-noise (S/N) ratio (to preserve the polarization state of the transmitted light) and high optical activity. Nonetheless, geometrically intrinsic reasons hinder the simultaneous demonstration of all these effects by single helical nanowires (SHN). Indeed, one of the main limiting factors for multifunctionality of SHNs consists of the loss of rotational symmetry determined by the end of the wire [20] , resulting in unwanted linear birefringence. This prevents obtaining broadband and high S/N ratio for circular polarizers [20] , and induces high sensitivity of the optical rotation to the structure orientation, thus limiting the potential applications of the device. Huge efforts in the fabrication of chiral metamaterial helices have been made to achieve several chiro-optical properties in only one structure. Tapered gold-helix metamaterials [21] were designed with direct laser writing to broaden the operation bandwidth in the THz region and reduce polarization intensity conversion [20] . Recently, using the focused ion beam-induced deposition (FIBID) technology, it has been possible to reach a broadband CD in the near-infrared optical region reducing the helix dimension to submicron size [22] . Wide band circular dichroic properties in the visible range were also demonstrated by planar stacked structures [15] , while 3D bichiral photonic crystals [23] , [24] , thought to limit the dependence of chiral effects on structure orientation, lead to the reduction of the infrared bandwidth. Rotational symmetry, intrinsically lacking in helix geometry, can be effectively restored with a packed multihelix arrangement in a single cell by the multihelical nanowire (MHN) configuration (similar to DNA strands), which have been recently theoretically proposed [20] , [25] , [26] , [27] , [28] . MHNs are predicted to operate as broadband circular polarizers in the visible range with high purity of circularly polarized transmitted light. However, the expected potentialities of MHN metamaterials have never been experimentally explored so far because of the absence of a suitable technology to face the challenges of realizing intertwined 3D complex structures with nanometre features as required for operation in the visible spectral region. Here we show the first realization of a triple-helical nanowire (THN) chiral metamaterial operating as highly pure broadband circular polarizers in the visible range, fabricated by a new nanotechnology method that combines the basic principles of tomography with the FIBID technique and that we named tomographic rotatory growth (TRG). The implemented technology allows the realization of complex and intertwined fully 3D structures such as THNs with nanoscale precision. According to the optical properties envisaged in previous theoretical work [20] , [25] , the realized THN samples enable optical multifunctionalities in the visible spectral range owing to the co-existence of intrinsic chirality and threefold rotational symmetry, namely giant broadband CD up to 37% and high S/N ratio (up to 24 dB) in the visible range (from 500 to 1,000 nm) because of the low light circular polarization conversion. Simultaneously, the fabricated THNs induce an optical rotation of the linearly polarized incident light up to 8°, as an effect of the only circular birefringence while the linear one is strongly suppressed (since the polarization rotation is largely independent from the sample orientation angle), underlining the ability of a high nanoscale polarization control. The developed TRG represents a viable method for the realization of new versatile miniaturized devices for nanophotonics, quantum optics and biological applications. Design and experimental realization The FIBID technique was already demonstrated to be a powerful tool for manufacturing 3D chiral structures at the nanoscale [22] ; however, the realization of intertwined helical structures by FIBID presents two additional technological challenges. One is the difficulty to extrude the nanowires in the third dimension because of the presence of blind spots (that is, the space occupied by the elements already grown). The other one is the extremely close distance of nanowires, introducing strong 3D mutual proximity effects, that prevent dimensional uniformity. These limiting factors were overtaken by developing the TRG method, in which the structure growth is stratified in multiple sections and combined with a split circular beam scan. In this growth mode, the basic scanning design (empty circle) is split into six arches arranged every 60° ( Fig. 1a ). The first fraction of the THN growth starts with the deposition of three platinum arches arranged every 120° (indicated in Fig. 1a with cyan colour and starting from the seeding sites 1, 3 and 5). The FIBID beam and pattern parameters were optimized following the procedure reported in ref. 22 , where is also described the dose compensation procedure used to strongly reduce the 3D proximity effects that, for the THN growth, was further implemented by using a continuous gradient function for dose correction. For the subsequent beam scan, the same pattern is repeated anticlockwise rotating by 60°, thus inducing the deposition of the arches arranged every 120° (indicated in Fig. 1a with magenta colour and starting from points 2, 4 and 6), completing one-third of a single helix revolution. For a complete THN loop, this procedure is repeated three times, as shown in the Supplementary Movie 1 . Structural continuity between consecutive arcs grown at different times during the circular beam motion is ensured by a careful calibration of pattern parameters that allows to match the seed cross-sectional area of the already grown arc. 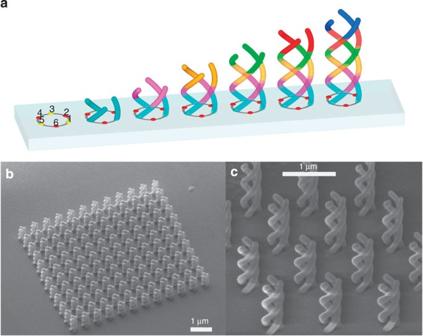Figure 1: Device fabrication. (a) Fabrication scheme to realize triple-helical nanowires (THNs). The basic two-dimensional layout consisting of an empty circle is divided in six sections (seeding sites arranged every 60°). During the first step, the circular motion of the beam leads to the 3D growth of three arches arranged every 120° (indicated with numbers 1, 3 and 5). Then, after changing the starting angle from 0° to 60° anticlockwise, the beam was moved to grow three arcs placed again every 120°. The extremely high level of alignment is achieved by setting the pattern parameters for a perfect overlap of consecutive arches. These two steps are repeated three times to get a complete loop of each subhelix. (b) SEM images of the array showing THNs with ED=375 nm, WD=110 nm and VP=705 nm. The THN array size is 10 μm × 10 μm, with lattice period=700 nm. (c) High-magnification image of a small array area evidencing the wire continuity and high dimensional uniformity of THNs in all three spatial directions obtained by the TRG method. Figure 1: Device fabrication. ( a ) Fabrication scheme to realize triple-helical nanowires (THNs). The basic two-dimensional layout consisting of an empty circle is divided in six sections (seeding sites arranged every 60°). During the first step, the circular motion of the beam leads to the 3D growth of three arches arranged every 120° (indicated with numbers 1, 3 and 5). Then, after changing the starting angle from 0° to 60° anticlockwise, the beam was moved to grow three arcs placed again every 120°. The extremely high level of alignment is achieved by setting the pattern parameters for a perfect overlap of consecutive arches. These two steps are repeated three times to get a complete loop of each subhelix. ( b ) SEM images of the array showing THNs with ED=375 nm, WD=110 nm and VP=705 nm. The THN array size is 10 μm × 10 μm, with lattice period=700 nm. ( c ) High-magnification image of a small array area evidencing the wire continuity and high dimensional uniformity of THNs in all three spatial directions obtained by the TRG method. Full size image Basically, the described method allows reducing a 3D complex geometry into a multiple planar structure formed by the image of subsequent sections of the 3D object, similar to what happens in tomography used for medical diagnostics. This approach, by solving the issue of blind spots for the ion beam, is also promising towards the development of a 3D printer at the nanoscale. The method validity is demonstrated by the THNs in Fig. 1b,c , where a perfect continuity of the wire helix is clearly shown. In Fig. 1b , the THN array formed by triple helices with external diameter (ED)=375 nm, single wire diameter (WD)=110 nm, vertical pitch (VP)=705 nm and distance between the centres of two adjacent helical wires of 235 nm is shown. The overall size of the THN array is 10 μm × 10 μm, with lattice period of 700 nm. The magnified scanning electron microscope (SEM) image of Fig. 1c shows the wire homogeneity and structural compactness of the THN array. The functional combination of 3D uniformity (by 3D proximity compensation), precise overlap among individual arcs (by pattern control) and the innovative fabrication method (TRG) has allowed the realization of THNs with highly controlled isotropy. The structure design resulted from finite difference time domain (FDTD) simulations as a function of the two main geometrical parameters, VP and ED ( Fig. 2 ), providing the best overlap between high extinction ratio (defined as T L / T R , amplitude contrast of the left circularly polarized (LCP) and right circularly polarized (RCP) transmissions, respectively) and broad circular dichroic bandwidth (defined as the wavelength range where the extinction factor values exceeded 1), in the visible spectral range. 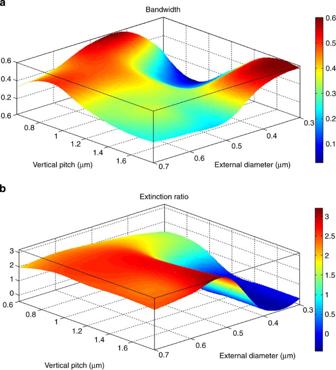Figure 2: Dichroic selectivity of triple-helical nanowires. Calculated dependence of THN circular dichroic properties on the two geometrical parameters (ED and VP): (a) bandwidth, (b) extinction ratio. A good combination of high extinction ratio and bandwidth is obtained for low values of VP (~600 nm) and external diameter ~400 nm. Figure 2: Dichroic selectivity of triple-helical nanowires. Calculated dependence of THN circular dichroic properties on the two geometrical parameters (ED and VP): ( a ) bandwidth, ( b ) extinction ratio. A good combination of high extinction ratio and bandwidth is obtained for low values of VP (~600 nm) and external diameter ~400 nm. Full size image Experimental characterization of chiro-optical effects The measured normal incidence transmittance and conversion spectra ( Fig. 3b ) of the square THN array (shown in Fig. 1b ) demonstrate a CD up to 37% ( Fig. 3c , solid line) with a broadband covering the wavelength range from 500 to 1,000 nm, in good agreement with the simulated CD ( Fig. 3c , dashed line). Reflection measurements performed for both LCP and RCP incident light reported in Supplementary Fig. 1 show very low values of reflection intensity allowing to assert that the losses in the transmission spectra are mainly related to the absorption mechanism that appears to be different for the two circular polarizations [29] . In Fig. 3d we report the spectrum of the S/N ratio, resulting ≥10 dB in the whole measured range, with maximum values of 24 dB reaching between 500 and 600 nm and two times larger than previously reported in SHNs [25] , [30] . 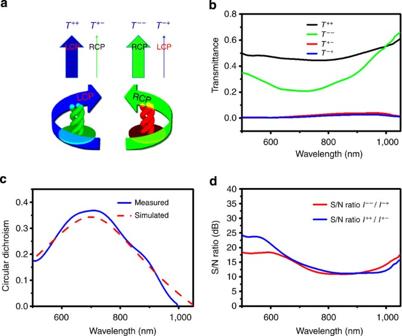Figure 3: Circular dichroism and signal-to-noise ratio. (a) Schematic representation to indicate the handedness of incident and transmitted circular polarization in the experimental measurements. (b) Measured transmission spectra (T++,T+−andT−−,T−+) for right circularly polarized (RCP) and left circularly polarized (LCP) incident light, respectively. (c) Measured (solid line) and simulated (dashed line) CD=(T++−T−−)/(T+++T−−), with peak value of 37% and broadband in the visible range. The simulated curve, obtained by varying the Pt content with dielectric function described by the Drude model, is calculated by considering an effective Pt content of 40%, as expected for the FIBID technique33. (d) Measured signal-to-noise (S/N) ratio, defined asI++/I+−(I−−/I−+). Figure 3: Circular dichroism and signal-to-noise ratio. ( a ) Schematic representation to indicate the handedness of incident and transmitted circular polarization in the experimental measurements. ( b ) Measured transmission spectra ( T ++ , T +− and T −− , T −+ ) for right circularly polarized (RCP) and left circularly polarized (LCP) incident light, respectively. ( c ) Measured (solid line) and simulated (dashed line) CD=( T ++ − T −− )/( T ++ + T −− ), with peak value of 37% and broadband in the visible range. The simulated curve, obtained by varying the Pt content with dielectric function described by the Drude model, is calculated by considering an effective Pt content of 40%, as expected for the FIBID technique [33] . ( d ) Measured signal-to-noise (S/N) ratio, defined as I ++ / I +− ( I −− / I −+ ). Full size image The wider band of THNs with respect to SHNs is not caused by nanostructure size dispersion as the THN presented consists of three identical and co-axial helices rotated by 120° with respect to each other. The mechanism inducing the dichroic band enlargement can be related mainly to mutual interaction between surface plasmon polaritons (SPP) mode excited by incident light in individual helical nanowires. In fact, the plasmon modes of the single nanowires, when combined in a THN configuration, start to interact, with a strength depending on the interwire separation and the radial penetration depth (1/ k ρ ) of the electromagnetic field associated with the SPP mode into the dielectric medium (air). At the frequency corresponding to the maximum CD value (700 nm), 1/ k ρ can be estimated [31] , [32] to be ~470 nm for pure platinum nanowires. Even considering a Pt/C mixture with 40% Pt and 60% C for the helical nanowires (which is the expected average Pt content of the investigated FIBID structures in agreement with the reported value for the FIBID technique in literature [33] ) this penetration length scales down to ~150 nm, that is, larger than the mutual interwire distance. In fact, because of the close-proximity arrangement of the helices, the air gap between the respective nanowires is only 100 nm. As a result, coupling and hybridization between the plasmon modes [34] of the intertwined nanowires is expected to occur, thus leading to a broader region of CD selectivity in the transmission spectra with respect to the SHN band ( Supplementary Fig. 2 ). Yang et al . theoretically explained with a similar mechanism the high S/N ratio expected in MHNs, being a parameter related to the current path generated on the helix wire surface by the interaction with the circularly polarized light [25] . The 120° spatial arrangement of THN leads to a threefold rotational symmetry allowing higher S/N ratio. On the contrary, the geometrical anisotropy of the SHNs is responsible for the partial transmission of the opposite light polarization, thus reducing the purity of the transmitted circularly polarized light. An additional property related to the complex geometry of THN structures is the ability to rotate the linear polarization state of the incident light. We performed the analysis of the optical rotatory dispersion (ORD) of the THN array through the experimental set-up schematically described in Fig. 4a . The longer axis of the transmitted polarization ellipse (induced by the sample dichroic properties) was used to measure the rotation of the polarization angle with respect to the linearly polarized incident light. The ORD was measured for different sample orientations, by rotating the sample ( Φ in ) in steps of 30°, as shown in Fig. 4c–h . 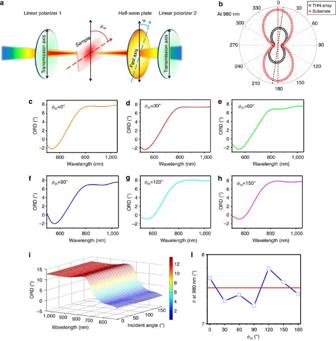Figure 4: Optical rotatory dispersion and circular birefringence. (a) Optical set-up scheme to measure optical rotatory dispersion (ORD) at different sample angles. Linearly polarized light transmitted by the sample is analysed with an half-wave plate cascaded with a second polarizer. The half-wave plate is rotated in steps ofα=2° with respect to the transmission axis of the linear polarizer, by means of a mechanically rotating stage, to obtain polar diagrams for the transmitted light intensity at each wavelength, similar to the one reported inbat 980 nm forΦin=0°. (c–h) Measured ORD at different sample angles by linearly polarized incident light. For each sample angle, the ORD shows similar trends, as expected by isotropic structures. (i) FDTD simulation of the ORD as a function of the input angle. The higher rotation value with respect to measurements is mainly related to the theoretical hypothesis of infinite array. (l) Optical activity measured in the crossing point (980 nm) where the linear polarization state is preserved. We note a very weak modulation (related to the extremely residual anisotropy of the nanostructures) around the mean value of 7.5° representing the polarization rotation only because of the circular birefringence. Figure 4: Optical rotatory dispersion and circular birefringence. ( a ) Optical set-up scheme to measure optical rotatory dispersion (ORD) at different sample angles. Linearly polarized light transmitted by the sample is analysed with an half-wave plate cascaded with a second polarizer. The half-wave plate is rotated in steps of α =2° with respect to the transmission axis of the linear polarizer, by means of a mechanically rotating stage, to obtain polar diagrams for the transmitted light intensity at each wavelength, similar to the one reported in b at 980 nm for Φ in =0°. ( c – h ) Measured ORD at different sample angles by linearly polarized incident light. For each sample angle, the ORD shows similar trends, as expected by isotropic structures. ( i ) FDTD simulation of the ORD as a function of the input angle. The higher rotation value with respect to measurements is mainly related to the theoretical hypothesis of infinite array. ( l ) Optical activity measured in the crossing point (980 nm) where the linear polarization state is preserved. We note a very weak modulation (related to the extremely residual anisotropy of the nanostructures) around the mean value of 7.5° representing the polarization rotation only because of the circular birefringence. Full size image The experimental results show the same trends for all Φ in angles with a polarization rotation of ~8° ( Fig. 4c–h ), corresponding to a specific rotatory power of 11,430° mm −1 (calculated as the maximum rotation angle normalized to the structure thickness). The same behaviour is shown by numerical simulations ( Fig. 4i ), which overestimate the rotation angle because of the theoretical assumption of an infinite array size. The strong ability to rotate the polarization axis of the light can be clearly evidenced by linearly polarizing the incident light, while a polarizer is placed at the output of the sample. In Fig. 5a,b we show the polarized light transmission images of the array. In the case of aligned-polarized light ( Fig. 5a ), transmitted light completely passes through the analyser only in the area surrounding the THN region while it is stopped at each single THN structure, resulting in a 6 × 6 array of dark (blue) dots corresponding to the THN positions. The inverse situation is obtained, in the case of cross-polarized light ( Fig. 5b ), with a 6 × 6 array of bright (red) dots on a dark background. 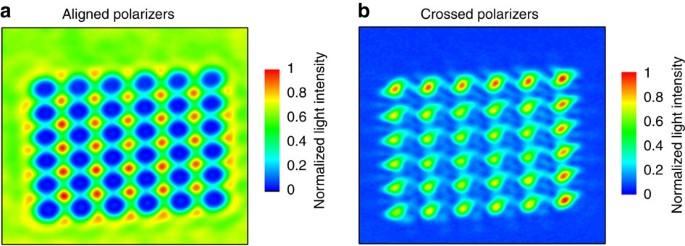Figure 5: Transmission maps of triple helical nanowire 6 × 6 array. (a,b) Transmission maps obtained with the microscope in polarized light configuration with a x 100 objective lens under normal incidence excitation. When the linear polarizer and the analyser are aligned, a bright-field image is created away from the THN region, while it appears darker in correspondence of each THN because of the circular birefringence effect (a). The situation is inverted when the analyser and the linear polarizer are crossed (b). Figure 5: Transmission maps of triple helical nanowire 6 × 6 array. ( a , b ) Transmission maps obtained with the microscope in polarized light configuration with a x 100 objective lens under normal incidence excitation. When the linear polarizer and the analyser are aligned, a bright-field image is created away from the THN region, while it appears darker in correspondence of each THN because of the circular birefringence effect ( a ). The situation is inverted when the analyser and the linear polarizer are crossed ( b ). Full size image Finally, we have analysed the polarization rotation angle ( θ ) dependence on the sample orientation ( Φ in ) at 980 nm, corresponding to the wavelength value with null dichroism, where a pure linear polarization rotation is expected. Figure 4j shows an average value of 7.5° for θ , corresponding to the measured optical activity induced only by the circular birefringence of the sample and related to the difference in the effective refractive index for the two circularly polarized components. The slight modulations (Δ θ <0.5°) around the average θ value provide a quantification of the residual anisotropy (revealing extremely weak linear birefringence) related to fabrication tolerances. We have presented a nanofabrication approach for manufacturing complex 3D nanostructures combining chiral and isotropic features. Such a TRG method applied to the FIBID technique enables the precise and continuous intertwining of multiple metal nanowires in a triple-helix configuration and can be further exploited for even more complex nanophotonic systems, paving the way towards the implementation of a 3D printer of nano-objects. To the best of our knowledge, this approach has allowed for the first time to experimentally demonstrate the unique combination of configurational properties exhibited by the THN metamaterial such as the co-existence of strong broadband CD with high conversion purity and optical activity, all in the visible range. The realized THNs can be employed in miniaturized optical components for chiral photonics, to fully control the light polarization state, towards the development of pure super achromatic polarization devices in the visible frequencies with applications in optoelectronic devices, integrated quantum optics, analytical chemistry, light-splitting systems, CD spectroscopy for biological detection and displays. THN fabrication The AlGaN/GaN/sapphire substrate was employed in the Carl Zeiss Auriga40 Crossbeam FIB/SEM system, equipped with the gas injection system. Trimethyl(methylcyclopentadienyl)-platinum (IV) precursor was locally injected on the sample. We optimized the injection distance between the substrate and nozzle and the scanning direction to obtain, respectively, high growth control by a suitable gas density, and high dimensional uniformity between nanohelices. The chamber pressure ranged from 1 × 10 −5 to 8 × 10 −6 mbar during the deposition time. To recover the pressure drop induced by effusion and the local depletion of the molecular density, we set a refresh time among single THNs. The growth strategy consists of splitting the basic layout into six arches rotated by 60° with respect to each other. The growth starts with the first three arches arranged every 120° with respect to the 0° angle and, after rotating the starting point by 60°, we grow the second three arches still arranged every 120°. This procedure is repeated for three times to obtain a full helix revolution. The nanostructure array (10 μm × 10 μm) is grown with ion beam current of 1 pA, accelerating voltage of 30 keV and step size of 10 nm. Experimental characterization All imaging of the nanostructure and the video in the Supplementary Movie 1 was performed using the FIB/SEM system in the coincidence point of the ion and electron beam. To quantify the CD in the chiral THNs, the transmission spectra were recorded in a confocal configuration by using a × 10 objective lens with numerical aperture (NA)=0.45 (ref. 22 ) under normal incidence illumination of a tungsten lamp. Circular polarization excitation was achieved using a combination of a linear polarizer and an achromatic quarter-wave plate. Light was focused on the sample by means of a condenser lens with NA<0.3. The microscope output image is collected and reconstructed on the entrance slits of a 200-mm spectrometer coupled to a CCD (charge-coupled device) camera for measurements in the visible range. The light transmission was calculated with respect to light transmitted by the unpatterned substrate. The S/N ratio is evaluated including in the set-up a second pair of linear polarizer and achromatic quarter-wave plate in the collection path to select both RCP and LCP transmissions for each incident light polarization state. The S/N ratio (dB) for each incident polarization is calculated as: with indicating the intensity of the transmitted YCP light when the incident beam is XCP (XCP and YCP indicate the left- (LCP) or right- (RCP) circular polarization of the incident and transmitted light, respectively, as shown in the equation 1). Finally, the ORD is measured by the same experimental set-up with linearly polarized incident light, while the transmitted light was analysed using an achromatic half-wave plate cascaded with a linear polarizer. The sample angle Φ in was rotated in steps of 30°, while the half-wave plate performed a 180° rotation in steps of 2° using a motorized stage. Numerical simulation The numerical simulations were performed using a commercial finite difference time-domain-based software (Lumerical FDTD Solutions). We defined the extinction factor as the ratio of the fundamental component of the transmission spectrum (corresponding to the far-field component) for left circular polarization and the corresponding spectrum for right circular polarization. According to this spectral function, for each configuration we evaluated the bandwidth from inside the larger 300- to 1,100-nm range of wavelengths, and where the extinction factor values exceeded 1 around the main peak resonance, the latter representing the most relevant footprint of the CD. For the calculation of the bandwidth and extinction factor, we set both the helix pitch and ED variable, leaving as fixed parameters the minimum THN-to-THN interstice in the squared array, the WD and the number of turns, which were set to 300, 110 and 1 nm, respectively. The THN-to-THN interstice values were chosen in order to obtain an effective filtering action avoiding strong THN-to-THN plasmonic resonances. The vertical pitch has been varied from 600 to 1,800 nm with a step of 20 nm, thus setting the internal pitch between contiguous branches of different subhelices to one-third of the total pitch. At the same time, the ED ranged from 300 to 700 nm with a step of 10 nm. A good combination of high extinction ratio and bandwidth is obtained for low values of VP (~600 nm) and ED ~400 nm. The slightly larger actual value of VP used for the fabricated THN (705 nm) was chosen to avoid connections among subhelices of THNs. The substrate has not been included in the simulations. How to cite this article: Esposito, M. et al . Triple-helical nanowires by tomographic rotatory growth for chiral photonics. Nat. Commun. 6:6484 doi: 10.1038/ncomms7484 (2015).